Experimental plug and play quantum coin flipping Performing complex cryptographic tasks will be an essential element in future quantum communication networks. These tasks are based on a handful of fundamental primitives, such as coin flipping, where two distrustful parties wish to agree on a randomly generated bit. Although it is known that quantum versions of these primitives can offer information-theoretic security advantages with respect to classical protocols, a demonstration of such an advantage in a practical communication scenario has remained elusive. Here we experimentally implement a quantum coin flipping protocol that performs strictly better than classically possible over a distance suitable for communication over metropolitan area optical networks. The implementation is based on a practical plug and play system, developed by significantly enhancing a commercial quantum key distribution device. Moreover, we provide combined quantum coin flipping protocols that are almost perfectly secure against bounded adversaries. Our results offer a useful toolbox for future secure quantum communications. Security is an imperative in all communication networks. Quantum communications hold the promise of achieving a security level that is impossible to reach by classical means. Indeed, information-theoretic security has been demonstrated for the task of distributing a secret key between two trusted and collaborating communicating parties using systems exploiting quantum effects [1] . However, many advanced cryptographic schemes belong to a model where the two parties do not trust each other and hence cannot collaborate. One of the fundamental primitives in this setting is coin flipping, in which two spatially separated distrustful parties share a randomly generated bit, whose value must be unbiased [2] . This functionality, either between two or more parties, is used in communication networks, for instance in online gaming and in randomized consensus protocols (due to its equivalence to the leader election functionality, a fundamental primitive in distributed computing) and is also an integral component for secure function evaluation [3] . When multiple parties are involved, coin flipping can be securely performed when more than half of the parties are honest. However, for two parties, which is the case that interests us here, we do not have such an honest majority. It is known that in the asynchronous classical model, perfectly secure coin flipping, that is, with a zero bias, is impossible without computational assumptions, while in the synchronous (or relativistic) model, unconditionally secure perfect coin flipping is possible [4] , at the expense of complex spatial configuration restrictions. Unfortunately, the impossibility result in the non-relativistic setting that we consider in this work holds even when protocols are enhanced with quantum communication [5] , [6] . A series of theoretical works, however, have demonstrated that the probability that an all-powerful malicious party can bias the coin, namely the cheating probability, can be strictly lower than 1 in the quantum setting, with an ultimate asymptotic bound of (refs 7 , 8 , 9 , 10 , 11 , 12 , 13 ). Moreover, a weaker version of coin flipping, which still remains useful for communication systems, can be almost perfectly achieved with quantum communication [14] , [15] . Coin flipping therefore provides a suitable framework to demonstrate an advantage of quantum over classical communication, achieving information-theoretic security in a non-cooperative model that is crucial for cryptographic applications beyond key distribution. To demonstrate such an advantage, we need to consider all imperfections that naturally appear in practical devices. For photonic systems, which constitute the chosen architecture for quantum communications, imperfections typically appear in the form of losses in the channel and measurement apparatus, and errors in the different implementation stages. Furthermore, systems suitable for long-distance communications over fibre-optic channels usually employ coherent light sources, thus becoming vulnerable to attacks exploiting the non-deterministic photon emission inherent in such sources [16] . Some of the aforementioned practical issues have been addressed in recent studies. An elegant solution to the problem of loss tolerance, that is, the tolerance to photon losses at any communication distance, was presented in ref. 17 , which however did not account for the presence of multiphoton pulses in coherent light source implementations. The cheating probability achieved by this protocol was slightly improved in subsequent work [18] , [19] . As a way to account for errors, the related primitive of bit string generation was also considered [20] , [21] , [22] . In practice, a first implementation concerned a protocol that becomes insecure for any loss [23] , while a promising solution gave results that unfortunately cannot be used in realistic conditions [24] . More recently, an implementation of the loss-tolerant protocol [25] used an entangled-photon source to eliminate the problem of multiphoton pulses. This was the first experiment that demonstrated an advantage of quantum over classical communication for coin flipping in the presence of losses and errors. However, although in principle the cheating probability bound in this protocol is independent of losses, a gain was shown in practice for a distance of a few metres. The closely related primitives of quantum bit commitment and oblivious transfer were experimentally demonstrated in the noisy storage model, where adversaries have access to an imperfect quantum memory [26] , [27] ; however, these protocols do not offer security against all-powerful adversaries. Finally, quantum bit commitment with relativistic constraints was also recently implemented [28] , [29] . Here, we provide a complete theoretical and experimental framework for the implementation of quantum coin flipping in practical communication scenarios. The protocol that we consider [30] takes standard experimental imperfections (multiphoton emission, transmission loss, detector inefficiency and dark counts) into account. We show that our protocol can be combined with protocols that achieve almost perfect security, that is, a bias asymptotically close to zero, against adversaries with bounded resources. More explicitly, if the adversary is bounded, then the protocol guarantees almost perfect security, while for an all-powerful adversary, the protocol still guarantees a security level strictly higher than classically possible. Providing security against adversaries of varying complexity is important in the context of current communication networks, where technological and computational capabilities can evolve very rapidly. Furthermore, we experimentally implement the protocol using a practical plug and play system, developed by significantly enhancing a commercial quantum key distribution (QKD) device ( http://www.idquantique.com ) [31] . The key element of our implementation is that we take a realistic approach: to account for the unavoidable errors in the system and for coherent light source emission statistics, we allow for a non-zero but small probability of abort when both parties are honest, and accept the dependence of the cheating probability on communication loss thus departing from absolute loss tolerance [17] , [25] . This constitutes an important change with respect to previous protocols and leads to a gain of three orders of magnitude in communication distance. Indeed, using a security analysis pertaining to our implementation and an appropriate benchmark for classical coin flipping protocols [32] , we can rigorously quantify the advantage offered by quantum communication as a function of distance, much in the way that the secret key fraction is calculated in QKD implementations [1] . In this way, we demonstrate a clear advantage for quantum coin flipping with information-theoretic security, at a communication distance suitable for metropolitan area network communications, with a system that can readily be deployed in such networks. Basic quantum coin flipping protocol The protocol that we analyse and implement in this work is schematically shown in Box 1 (ref. 30 ). Alice sends to Bob a fixed number K of photon pulses in states , each of which is prepared independently following a uniformly random choice of basis α i and bit c i , with i =1,…, K , and a fixed protocol parameter y (see Supplementary Fig. 1 for a description of the states). Bob measures the K pulses by selecting uniformly at random bases β i , and replies with the position of the first successfully measured pulse j and a random bit b . Alice then reveals the basis and the bit used for that position: if the bases of the two parties agree, but the measurement output of Bob is not the same as Alice’s bit, they abort. In all other cases, they agree that the coin value is c j ⊕ b . A crucial feature of the protocol is the assumption that the states are generated by an attenuated coherent light source, which is a standard element of practical implementations. Therefore, each pulse contains a number of photons that follows a Poisson distribution with mean photon number μ . Standard experimental imperfections are accounted for by introducing a probability to abort even when both parties are honest. This probability, denoted H , is determined by the experimental parameters, namely the mean photon number per pulse μ , the number of protocol rounds K , the channel length, the detector quantum efficiency and dark count rate and the error rate. Then, optimal cheating strategies for an all-powerful malicious party can be devised for both Alice and Bob, leading to expressions for the maximal cheating probabilities, and , respectively (see Supplementary Note 1 for details). These are functions of μ and K , hence for a given desired honest abort probability, it is possible to minimize the cheating probabilities by finding optimal values for these parameters. In addition, the parameter y can be appropriately adjusted so that , which means that the protocol is fair. This analysis allows us to evaluate the maximal cheating probability attained for any given honest abort probability, for different communication distances. A security analysis allowing for a non-zero honest abort probability has also been performed for classical coin flipping protocols [32] , providing the cheating probability bound , for H <1/2, which is the honest abort probability region of practical interest. This can be used as a benchmark to assess quantitatively the advantage offered by the use of quantum resources for coin flipping. Box 1: Basic quantum coin flipping protocol. Experimental setup We perform the demonstration of our quantum coin flipping protocol using a plug and play system, which is a considerably enhanced version of the commercial system Clavis 2 of ID Quantique, designed for QKD. The experimental setup, shown in Fig. 1 , employs a two-way approach: light pulses at 1550, nm are sent from Bob to Alice, who uses a phase modulator to encode her information. The pulses are then reflected by a Faraday mirror and attenuated to the desired level before being sent back to Bob. Finally, Bob chooses a measurement basis with his phase modulator and registers the detection events using two high-quality single-photon detectors. When the BB84 QKD protocol [33] is implemented by the plug and play system, the states prepared by Alice and measured by Bob correspond to the states used in our quantum coin flipping protocol, with y =1/2. Hence, the quantum transmission stage of the QKD protocol is identical to that of the coin flipping protocol with the exception that, in the latter, y should be appropriately modified to guarantee the fairness of the implemented protocol. In practice, this parameter is set using the control signal that drives Alice’s phase modulator, which is also used to encode Alice’s basis and bit information. 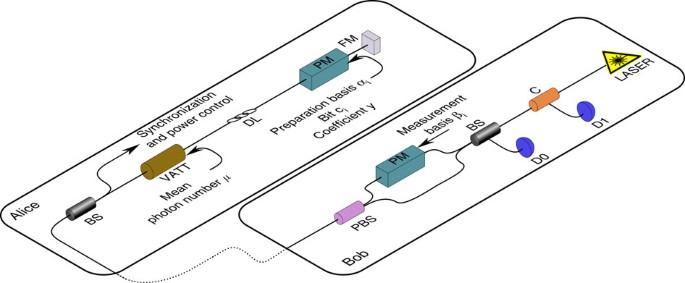Figure 1: Experimental setup of the plug and play system. The laser source at Bob’s setup emits photon pulses at 1,550 nm, which are separated at a 50/50 beam splitter and then recombined at a polarization beam splitter, after having travelled through a short and a long arm. The latter contains a phase modulator and is appropriately arranged to transform horizontally polarized to vertically polarized states and vice versa. The pulses then travel to Alice through the communication channel, are reflected on a Faraday mirror, appropriately modulated and attenuated and travel back to Bob orthogonally polarized. As a result, the pulses now take the other path at Bob’s side and arrive simultaneously at the beam splitter, where they interfere. Finally, they are detected by two InGaAs avalanche photodiode (APD) single-photon detectors. To implement the quantum coin flipping protocol, Alice chooses her basis and bit values by applying a suitable phase shift to the second pulse with her phase modulator. This modulator is also used to apply the state coefficienty. She also uses her variable attenuator to apply the required attenuation for a desired mean photon number per pulseμ. Bob chooses his measurement basis by applying an appropriate phase shift at the first pulse on its way back using his phase modulator. This interferometric setup compensates for all fluctuations in the channel, which guarantees an excellent system stability. BS, beam splitter; C, circulator; D0,D1, APD detectors; DL, delay line; FM, faraday mirror; PBS, polarization beam splitter; pm, phase modulator; VATT, variable attenuato. Figure 1: Experimental setup of the plug and play system. The laser source at Bob’s setup emits photon pulses at 1,550 nm, which are separated at a 50/50 beam splitter and then recombined at a polarization beam splitter, after having travelled through a short and a long arm. The latter contains a phase modulator and is appropriately arranged to transform horizontally polarized to vertically polarized states and vice versa. The pulses then travel to Alice through the communication channel, are reflected on a Faraday mirror, appropriately modulated and attenuated and travel back to Bob orthogonally polarized. As a result, the pulses now take the other path at Bob’s side and arrive simultaneously at the beam splitter, where they interfere. Finally, they are detected by two InGaAs avalanche photodiode (APD) single-photon detectors. To implement the quantum coin flipping protocol, Alice chooses her basis and bit values by applying a suitable phase shift to the second pulse with her phase modulator. This modulator is also used to apply the state coefficient y . She also uses her variable attenuator to apply the required attenuation for a desired mean photon number per pulse μ . Bob chooses his measurement basis by applying an appropriate phase shift at the first pulse on its way back using his phase modulator. This interferometric setup compensates for all fluctuations in the channel, which guarantees an excellent system stability. BS, beam splitter; C, circulator; D0,D1, APD detectors; DL, delay line; FM, faraday mirror; PBS, polarization beam splitter; pm, phase modulator; VATT, variable attenuato. Full size image Alice sets the average photon number per pulse μ with the variable attenuator shown in Fig. 1 , using a previously established calibration relationship. It is important to note that typical uses of the Clavis 2 for QKD employ significantly higher μ values. In Methods, we provide a comprehensive description of the crucial improvements made on the system to allow it to perform quantum coin flipping, which also included an appropriate adjustment of the calibration and synchronization procedures. At the end of the quantum transmission part of the protocol, we derive a set of data containing the preparation and measurement basis choices of Alice and Bob, respectively, and the measurement outcomes of Bob, similarly to the raw key data obtained in QKD experiments. Security of the implementation The security proof of the basic quantum coin flipping protocol provided in ref. 30 takes into account standard experimental imperfections (multiphoton emission, transmission loss, detector inefficiency and dark counts), which are present in our system. This analysis, however, is based on the following three important assumptions, whose validity has to be carefully examined for our implementation: (i) Honest Alice can create each state with equal probability and independently of Bob; (ii) For the first pulse j that honest Bob successfully measures, his basis β j and bit b are uniformly random and independent of Alice; (iii) For the first pulse j that honest Bob successfully measures and for any state that Alice sends and any basis that Bob measures, the probabilities that Bob obtained a specific outcome are exactly proportional to the squares of the projection of Alice's state to each basis vector. Even though these assumptions are routinely made in theoretical security proofs, they do not necessarily hold in practice unless extra caution is taken. For example, when Alice creates her states via an entangled-photon source, by measuring one half of the entangled pair and sending the other half to Bob, then the probabilities of creating each state will depend on the individual efficiencies of the detectors she uses for her measurement. Similarly, when Bob performs a measurement using a high-efficiency detector for the outcome 0 and a lower-efficiency one for 1, then there is a bias of his outcome that Alice may use to her advantage. Last, if a different set of detectors is used for each of the two bases, again Bob's probability of successfully measuring in one basis may be much greater than in the other one. In this case, Alice can increase her cheating probability by revealing the latter basis with higher probability, thus forcing Bob to accept with higher probability. Let us now discuss how it is possible to ensure that the aforementioned assumptions are satisfied in our implementation. Assumptions (i) and (ii), which concern Alice’s choice of states and Bob’s choice of measurement bases and bit b , respectively, can be addressed in a similar way. Alice uses a quantum random number generator to pick the basis and bit that define her state, and applies the selected phase shift using her phase modulator. Similarly, Bob uses his quantum random number generator to generate his bit b and to pick the measurement basis, which is followed by the corresponding phase shift applied by his phase modulator. Therefore, in both cases, possible deviations from the uniform distribution can result from the bias of the quantum random number generators and the variation in the capability of the phase modulators to apply different phase shift values. These effects are expected to be quite small; indeed, this is confirmed by extensively analysing the data obtained from our experimental setup and deriving appropriate bounds for these deviations (see Supplementary Note 1 for details). Assessing assumption (iii), which concerns Bob’s basis and outcome distributions given a detection event, turns out to be particularly important. We would like to ensure that when Bob has registered a detection this happens on each one of the two bases with uniform probability. In our experimental setup, the same set of detectors is used for both bases so we do not expect an important deviation from a uniform distribution, which is again confirmed by our data. However, we observe a significant asymmetry in the number of detections registered by each detector; in fact, the ratio of the detection efficiencies is found to be approximately 0.68 (see Supplementary Table 1 ). This asymmetry can clearly be used by malicious Alice to increase her cheating probability. To remedy this problem, we implement a simple yet powerful solution proposed in ref. 26 , the symmetrization of losses. Bob effectively makes the detection efficiencies equal by throwing away some detection events from the detector featuring higher efficiency. Even after this symmetrization procedure, an uncertainty on the efficiency ratio remains and can be appropriately bounded. In Supplementary Note 1 , we provide a rigorous security analysis of the basic quantum coin flipping protocol, when it is implemented using a practical plug and play system. This analysis takes into account all standard imperfections, as well as the additional inevitable imperfections present in our system that were previously discussed, and is used to derive the cheating probabilities that are necessary to assess quantitatively the advantage offered by quantum communication for coin flipping. This procedure is performed using several values of μ for each channel length, and then choosing the number of rounds K to attain the desired honest abort probability. On the basis of these sets of parameters, we derive the cheating probabilities of a malicious Alice and Bob, and , respectively, using the extended security analysis of the basic quantum coin flipping protocol (see Supplementary Note 1 for the full expressions). This allows us to find, for both channel lengths, the sets of values for μ , K and y that minimize the cheating probability and at the same time make the protocol fair . Note that for simplicity, the y values of our experimental data have been chosen independently of the honest abort probability value; in practice, slight modifications of these values might be required to achieve a perfectly fair protocol for each specific honest abort probability. The optimized experimental parameters for an honest abort probability H =0.8% are shown in bold in Table 1 . Table 1 Experimental parameter values for H =0.8%. Full size table In Fig. 2 we show the cheating probability calculated from our experimental data for 15 and 25 km, as a function of the honest abort probability. For each value of the honest abort probability, the number of rounds K and mean photon number per pulse μ has been optimized as explained previously. The uncertainty in the estimation of μ is illustrated by the shaded areas in the plot. To quantify the advantage offered by quantum communication, we use the classical cheating probability bound, p c (ref. 32 ). We can see that the cheating probability is strictly lower than classically possible for a distance of 15 km, for a wide range of practical values of the honest abort probability. In particular, taking into account finite-size effects, for a range of honest abort probability from 0.4 to 1.45%, the cheating probability is lower than classically possible unless with probability of the order 10 −9 . The area corresponding to the data obtained at 25 km is just above the classical cheating bound for all honest abort probability values, which means that a quantum advantage cannot be claimed in this case. 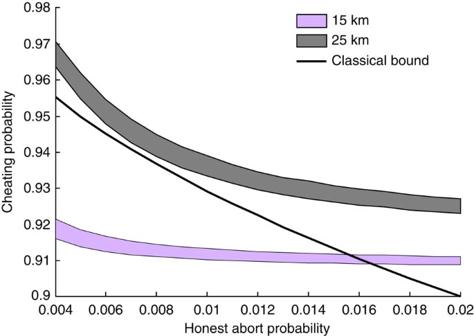Figure 2: Cheating versus honest abort for 15 and 25 km. The cheating probability for each honest abort probability value is calculated from the experimental data using the security analysis of the basic quantum coin flipping protocol adapted to our implementation. The values correspond to a fair protocol. The shaded areas are derived from the uncertainty in the estimation of the average photon number per pulse exiting Alice’s setup. The solid line represents the cheating probability bound for classical coin flipping protocols. For a 15 km channel length, quantum communication leads to lower cheating probability values than is classically possible, for a wide range of practical honest abort probabilities. The cheating probabilities derived at 25 km are always greater than the classical bound. Figure 2: Cheating versus honest abort for 15 and 25 km. The cheating probability for each honest abort probability value is calculated from the experimental data using the security analysis of the basic quantum coin flipping protocol adapted to our implementation. The values correspond to a fair protocol. The shaded areas are derived from the uncertainty in the estimation of the average photon number per pulse exiting Alice’s setup. The solid line represents the cheating probability bound for classical coin flipping protocols. For a 15 km channel length, quantum communication leads to lower cheating probability values than is classically possible, for a wide range of practical honest abort probabilities. The cheating probabilities derived at 25 km are always greater than the classical bound. Full size image To obtain further insight into our results, we define a gain function, as follows: where p c and p q are the classical cheating probability bound and the quantum cheating probability value derived from our experimental data, respectively. If the experimental data yields a positive G for a certain honest abort probability, this means that these results cannot be obtained by any purely classical means. We can then use the gain as a figure of merit to assess the performance of our quantum coin flipping implementation in a secure communication scenario. In Fig. 3 , we show the gain as a function of distance, for a fixed honest abort probability H =0.8%. For the channel length of 15 km, a distance which is sufficient for many applications requiring communication over metropolitan area networks, the gain is about 0.025, while for the channel length of 25 km no positive gain can be obtained. 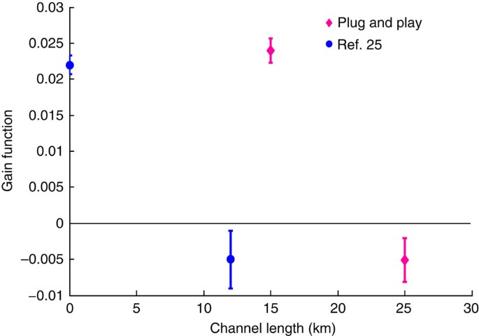Figure 3: Gain as a function of channel length. The gain function is calculated as the difference between the classical and quantum cheating probability, and illustrates the advantage offered by the use of quantum communication for coin flipping. The uncertainty in the gain function comes from the error in estimating the average photon number per pulse in Alice’s setup. The diamonds correspond to the cheating probabilities achieved by our plug and play implementation for 15 and 25 km, for a fixed honest abort probability of 0.8%. A positive gain is obtained for 15 km, while the gain remains below the classical limit for 25 km. For comparison, previous experimental results based on an entangled-photon source implementation of a loss-tolerant quantum coin flipping protocol25are also shown (circles): a positive gain was experimentally obtained for a distance of 10 m, with an honest abort probability of 1.8%, while no positive gain was possible for a distance of 12 km. Figure 3: Gain as a function of channel length. The gain function is calculated as the difference between the classical and quantum cheating probability, and illustrates the advantage offered by the use of quantum communication for coin flipping. The uncertainty in the gain function comes from the error in estimating the average photon number per pulse in Alice’s setup. The diamonds correspond to the cheating probabilities achieved by our plug and play implementation for 15 and 25 km, for a fixed honest abort probability of 0.8%. A positive gain is obtained for 15 km, while the gain remains below the classical limit for 25 km. For comparison, previous experimental results based on an entangled-photon source implementation of a loss-tolerant quantum coin flipping protocol [25] are also shown (circles): a positive gain was experimentally obtained for a distance of 10 m, with an honest abort probability of 1.8%, while no positive gain was possible for a distance of 12 km. Full size image Note that in the distrustful model with information-theoretic security, it is not known if it is possible for Alice and Bob to collaborate in order to increase the robustness of the implementation. This results in an inherent limitation to the attainable communication distance in our quantum coin flipping implementation. However, the use of better single-photon detectors with lower dark count rates [34] for instance, can readily extend the range of our protocol. Finally, in our implementation, the classical steps of the coin flipping protocol following the quantum transmission are not performed in real time. However, it is clear that the coin flipping rate will be dominated by the time that it takes for K pulses to travel from Alice to Bob. For a laser pulse repetition rate of 10 MHz, this corresponds roughly to a few tens of coin flips per second. As we can see in Table 1 , if Alice increases the average photon per pulse exiting her system, the required number of protocol rounds reduces, which also reduces the runtime for the protocol, but this comes at the expense of a slightly higher cheating probability. Again, using better single-photon detectors can result in a substantially lower number of required rounds. In a real communication scenario of two distrustful parties wishing to agree on a coin value using the plug and play system, the parties would be given a choice of gain values for a range of honest abort probabilities given their communication distance and the desired communication rate. Enhancing security against bounded adversaries We have seen that our basic quantum coin flipping protocol achieves information-theoretic security, which is impossible classically. However, this security level comes at a price of a high bias; indeed, as we see in Fig. 2 , the unbounded adversary can bias the coin with probability greater than 90%. This might not be suitable for some applications. It is then interesting to consider combining our protocol with protocols that achieve a bias asymptotically close to zero against bounded adversaries. Combining protocols with different types of security is in fact a powerful concept, which is widely used in practice. This allows communications to remain secure not only at the present time but also in the future, accommodating at the same time for different types of adversaries with unknown or rapidly evolving technological and computational capabilities. To construct combined protocols for quantum coin flipping, we apply the following general lines: We discern three stages, as in the commonly used protocols against bounded adversaries, including classical protocols employing one-way functions [3] and quantum protocols in the noisy quantum storage model [26] , [35] . In the first stage (commit), which remains unchanged from the protocols against bounded adversaries, Alice and Bob exchange classical or quantum messages such that at the end of this stage each party has almost perfectly committed to one bit, S and T , respectively. In the second stage (encrypt), Alice and Bob encrypt their respective random bits using the committed values. In particular, Alice sends K pulses using the states , for i =1,…, K , and Bob replies by sending T ⊕ b as well as j , the index of the first measured pulse, as in the basic protocol. In the third stage (reveal), Alice and Bob reveal ( c j , S ) and ( b , T ), respectively, together with additional information depending on the underlying bounded adversary model and, if nobody aborts, the value of the coin is c j ⊕ b (see Supplementary Note 2 for explicit combined protocols for models with computationally bounded adversaries and adversaries with noisy quantum storage). The combined protocols constructed as explained above achieve an almost perfect security against bounded adversaries, exactly as the original protocols; in addition, when the adversaries are unbounded, they still cannot cheat with a probability higher than the one provided by our basic quantum coin flipping protocol, which is strictly better than classically possible. Hence, these protocols offer the maximal possible security guarantees. The results that we have presented constitute one of the few instances of a rigorously proven and demonstrated advantage of quantum over classical communication, which can be used for practical secure communications between distrustful parties with information-theoretic security guarantees. We have demonstrated this advantage using a practical plug and play system over distances suitable for metropolitan area communication networks. This enlarges the scope of quantum cryptography, in particular to practical applications where the parties do not trust each other. We emphasize that dealing with distrustful parties is more complicated than the QKD scenario, both in theory and in practice. For example, although randomized procedures like error correction and privacy amplification that are widely employed in QKD have been used in the security analysis of protocols dealing with bounded adversaries [36] , it is an open question whether such procedures can be used in the information-theoretic security setting; in principle, any such step can be used by the malicious party to his or her advantage. Therefore, new techniques may be needed in order to deal with the imperfections of the implementation and the inherent limitations to the attainable communication distance. Our results bring quantum cryptography in the distrustful model at a comparable level of practicality as QKD and provide means to benchmark this type of primitives in a way similar to QKD protocols. In addition, by combining our quantum coin flipping protocol with protocols secure against bounded adversaries we enhance those with a level of information-theoretic security. This assures that an honest party will always obtain security guarantees stronger than possible by classical means. It is also interesting to note that our protocol is based on a bit commitment scheme, augmented only by an additional classical message from Bob to Alice between the commit and reveal stages. This means that our combined coin flipping protocols can also be viewed as commitment schemes where both parties commit some value to each other. Hence, our security analysis can be extended in a straightforward way to hold for bit commitment in the computational models that we have considered. In the same way, our implementation indeed performs plug and play quantum bit commitment. We also note that a weaker, but still very powerful, variant, called weak coin flipping, with almost perfect information-theoretic security is in theory possible with quantum technology [14] , [15] . Our implementation is a first step towards making such protocols a reality, however the quantum protocols that achieve almost perfect security are not well understood and currently necessitate large-dimension entangled states. Simplifying such protocols is an important open question. Last, as in practical QKD, our implementation of quantum coin flipping may be vulnerable to side-channel attacks (see Methods for details). The power control setup placed at the entrance of Alice’s system as a countermeasure for the so-called Trojan horse attacks [37] can also be used by Alice to properly characterize the photon distribution of the pulses sent by Bob [38] . This is important to counter, for instance, an attack by which Bob sends strong light pulses to Alice, which lead to an increased average photon number per pulse and consequently to a greater cheating probability. Identifying potential side-channel attacks and devising appropriate countermeasures is of great importance, as for all practical quantum cryptographic systems. Plug and play quantum coin flipping system Our quantum coin flipping implementation is based on the commercial QKD system Clavis 2 of ID Quantique. Using a QKD system for an implementation of a cryptographic primitive that requires an entirely different security analysis and operates in non-standard experimental conditions necessitated several important modifications to the system. First, single-photon detectors with very low dark count rates were installed in the quantum coin flipping system; indeed, the honest abort probability is very sensitive to this parameter and so with even moderately high dark counts the quantum advantage vanishes at any distance. The dark count rates per detection gate of the detectors D 0 and D 1 were 7 × 10 −6 and 1.6 × 10 −6 , with corresponding quantum efficiency values of 7.7% and 5.2%, respectively. Second, new functionalities and control signals were added to the system to be able to apply the coin flipping protocol, in particular, those allowing us to rotate the standard BB84 states so that the optimal states for a fair protocol could be used and those allowing us to reduce the mean photon number per pulse μ at suitable values for coin flipping. These values were in fact one or two orders of magnitude lower than those typically used for QKD. This last point was also crucial for many aspects of the implementation, as a very low μ value hindered the operation of several embedded calibration and testing processes of the system, which were therefore entirely redesigned. Such calibration procedures play an important role in the two-way configuration of the plug and play system, which imposes particular care in the synchronization of the phase shift and attenuation signals, and the detection gates. Among those, of particular importance is the calibration procedure involving the variable attenuator at Alice’s site, which was actually the main source of the uncertainty that we observe in our data. Finally, the QKD classical post-processing procedures were replaced by our software, which used as an input the raw data of quantum signal exchange between Alice and Bob, together with basis choice information. These enhancements led to the development of a practical, plug and play system that is capable of performing quantum coin flipping in addition to key distribution. It is important to note that the advantage of the plug and play system with respect to other systems providing the functionalities required by our protocol is that it offers a particularly robust and stable implementation, which allows to perform experiments at low signal level for long time duration, resulting in very reliable results. This system can also potentially be used for protocols employing decoy states [39] , [40] , [41] . Although the use of decoy states is a powerful tool for achieving practical long-distance QKD and for improving the performance of quantum cryptographic protocols in the noisy storage model [36] , it is not known, to the best of our knowledge, if a protocol employing decoy states can be devised for quantum coin flipping providing security against all-powerful adversaries. Side channels and practical security Our quantum coin flipping implementation takes explicitly into account the standard imperfections (multiphoton emission, transmission loss, detector inefficiency and dark counts) present in practical systems. We also consider imperfections related to asymmetries in the detection efficiency and basis-dependent flaws in the components of Alice’s and Bob’s devices, which play a crucial role for the practical security of the implementation. It is clear, however, that similarly to QKD experiments, further deviations between the security proof and the actual implementations inevitably exist and can lead to side-channel attacks by the adversary. Although an exhaustive analysis of possible side channels is out of the scope of the present work, we examine a few prominent cases known in the context of QKD demonstrations, some of which are particularly relevant for the plug and play system at the basis of our implementation. In the setting of QKD, an efficient eavesdropping attack that also applies to the plug and play system consists in shifting in time the second pulse (see Fig. 1 ) such that this pulse is only partially modulated by Alice’s phase modulator. This so-called phase remapping attack [42] , [43] effectively alters the relative phase between the two pulses and allows Eve to obtain key information for ranges of quantum bit error rate values that would otherwise be considered acceptable. In the distrustful setting of quantum coin flipping, malicious Bob attempts to maximize his cheating probability by performing an optimal measurement to the received states, and so reducing the probability of distinguishing them cannot help him. In addition, errors in the state preparation performed by Alice have been considered in detail in the security analysis of our implementation (see Supplementary Note 1 ). Similarly, attacks exploiting the loophole introduced by detection efficiency mismatch, such as the time-shift attack [44] , [45] , [46] , are, in principle, excluded by the symmetrization procedure included in our experimental protocol. Finally, an effective countermeasure against the powerful blinding attack [47] , where the single-photon detectors are brought to a classical operation regime and can be fully controlled by the adversary, consists in randomly suppressing detector gates and emitting an alarm signal in case of registered detection events during those gates. This countermeasure is implemented in our system. In addition to the aforementioned side-channel attacks, it is important to note the issue of phase randomization [48] , which is an assumption typically made in security proofs and hence should be satisfied in practice. Phase randomization together with suitable intensity monitoring are also required for the characterization of an untrusted source, which is particularly relevant for the plug and play system [38] . Although all the hardware components necessary for implementing active phase randomization and source characterization at Alice’s site are available in our system, these processes were not performed in real time, mainly due to the difficulty in generating random real numbers in real time and to the limited bandwidth of the threshold discriminator used for intensity monitoring. Clearly, for any real-life implementation, following such procedures is essential. How to cite this article: Pappa, A. et al. Experimental plug and play quantum coin flipping. Nat. Commun. 5:3717 doi: 10.1038/ncomms4717 (2014).